Cretaceous stem chondrichthyans survived the end-Permian mass extinction Cladodontomorph sharks are Palaeozoic stem chondrichthyans thought to go extinct at the end-Permian mass extinction. This extinction preceded the diversification of euselachians, including modern sharks. Here we describe an outer-platform cladodontomorph shark tooth assemblage from the Early Cretaceous of southern France, increasing the fossil record of this group by circa 120 million years. Identification of this material rests on new histological observations and morphological evidence. Our finding shows that this lineage survived mass extinctions most likely by habitat contraction, using deep-sea refuge environments during catastrophic events. The recorded gap in the cladodontomorph lineage represents the longest gap in the fossil record for an extinct marine vertebrate group. This discovery demonstrates that the deep-sea marine diversity, poorly known during most of the fish evolutionary history, contains essential data for a complete understanding of the long-term evolution of marine fish paleobiodiversity. The fossil record of coelacanths, or actinistians, is characterized by a gap of circa 70 million years (myrs) preceding the living Latimeria and shows a constriction of habitats from all platform environments in the Late Cretaceous to mesobenthic in modern environments. Coelacanths survived the Cretaceous/Palaeogene mass extinction probably by occupying deep-sea environments as a refuge [1] . Similar to the Cretaceous/Palaeogene boundary, the Permian/Triassic boundary marks a sharp turnover within fish groups and chondrichthyans in particular [2] , with marine Palaeozoic stem chondrichthyans (for example, cladodontomorphs, petalodontiforms, bransonelliforms, eugeneodontiforms) being replaced by hybodont sharks and modern elasmobranchs. Here we report a cladodontomorph shark assemblage including minute-size dental remains obtained by bulk sampling of an indurate limestone bed corresponding to relatively deep outer platform deposits [3] from the Valanginian (Early Cretaceous, 139.8–132.9 myrs ago) of southern France. Tooth morphologies and enameloid microstructure features indicate that the three fossil taxa described here belong to the Cladodontomorphii, a Palaeozoic stem chondrichthyan group thought to vanish at the end-Permian. The presence of cladodontomorph sharks in Valanginian outer-platform deposits increases the fossil record of this group by circa 120 myrs and provides new insights in the evolutionary history of this clade, which shares similar features with the last 70 myrs of evolutionary history of coelacanths. This discovery suggests that relatively deep-sea habitats served as refuge for representatives of some ancient fish lineages and shows that the scarcity of deep-sea deposits yielding vertebrate remains obscures large parts of the evolution of marine vertebrate palaeobiodiversity. Geological setting The sampled sedimentary succession corresponds to Berriasian and Valanginian marine argillaceous limestones and marls, the remaining Early Cretaceous succession being lacking owing to a marked regression and corresponding erosion. The sampled site ( Fig. 1 ) is situated 7 km east to the town of Ganges (North of Montpellier) close to a farm named ‘Mas d'Antrigoule’ (Gard County). In this area, the Early Valanginian sedimentary unit reaches a thickness of 150–200 m and corresponds to outer platform deposits (see ref. 3 for detailed invertebrate faunal list) marked by sedimentary perturbations (for example, sediment slumps) on the western side of the Vocontian Basin. This sedimentary unit is composed of finely stratified calcareous marls with intercalated decimetric argillaceous limestone beds. The sampled elasmobranch-rich horizon is an indurate hardground of about 20 cm thick including numerous bioclasts and worm tubes. The Valanginian age of this horizon is attested, among others, by the presence of Neocomites neocomiensis, whereas upper in the formation, the presence of Eristavites indicates the very base of the Late Valanginian [3] . Thus, the sampled horizon can be considered latest early Valanginian in age. Reworking of the fossils from Palaeozoic rocks is ruled out because teeth (especially the roots) are extremely fragile but well preserved and because no non-metamorphized (Hercynian episode) Palaeozoic marine strata crop out in the region. 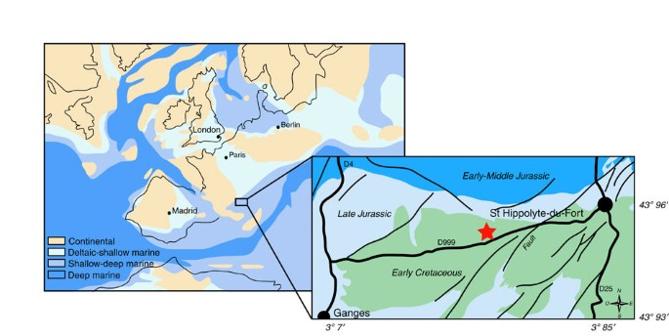Figure 1: Early Cretaceous palaeogeographic setting of Europe. Enclosed: close-up on the sampled site (red star) with surrounding geological units. Figure 1: Early Cretaceous palaeogeographic setting of Europe. Enclosed: close-up on the sampled site (red star) with surrounding geological units. Full size image Systematic palaeontology The systematic framework used here follows that of Ginter et al. [4] , whereas Cappetta [5] is followed for terminology. Class Chondrichthyes Huxley, 1880 Superorder Cladodontomorphii Ginter, Hampe and Duffin, 2010 Order Symmoriiformes Zangerl, 1981 Family Falcatidae Zangerl, 1990 Falcatidae indet. ( Fig. 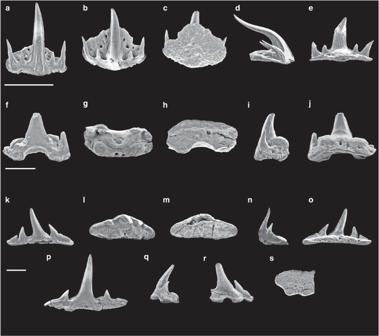Figure 2: Cladodontomorph shark teeth recovered from the Valanginian of southern France. (a–e) Falcatidae indet., VAL 36, tooth in (a) labial, (b) occlusal, (c) basal, (d) profile and (e) lingual views. Scale bar, 500 μm. (f–j) Ctenacanthiformes indet. VAL 54, tooth in (f) labial, (g) occlusal, (h) basal, (i) profile and (j) lingual views. Scale bar, 500 μm. (k–s) Cladodontomorphii indet. (k–o) VAL 55, tooth in (k) labial, (l) occlusal, (m) basal, (n) profile and (o) lingual views. (p) VAL 56, tooth in labial view. (q–s) VAL 57, tooth in (q) profile, (r) labial and (s) basal views. Scale bar, 500 μm. 2a–e ) Figure 2: Cladodontomorph shark teeth recovered from the Valanginian of southern France. ( a – e ) Falcatidae indet., VAL 36, tooth in ( a ) labial, ( b ) occlusal, ( c ) basal, ( d ) profile and ( e ) lingual views. Scale bar, 500 μm. ( f – j ) Ctenacanthiformes indet. VAL 54, tooth in ( f ) labial, ( g ) occlusal, ( h ) basal, ( i ) profile and ( j ) lingual views. Scale bar, 500 μm. ( k – s ) Cladodontomorphii indet. ( k – o ) VAL 55, tooth in ( k ) labial, ( l ) occlusal, ( m ) basal, ( n ) profile and ( o ) lingual views. ( p ) VAL 56, tooth in labial view. ( q – s ) VAL 57, tooth in ( q ) profile, ( r ) labial and ( s ) basal views. Scale bar, 500 μm. Full size image Material. One tooth (specimen VAL 36). Locality, horizon and age. Mas d’Antrigoule, (Gard County, Southern France); N. neocomiensis Zone, latest early Valanginian (Early Cretaceous). Description This unique tooth is composed of an elongate and slender main cusp strongly oriented lingually and sigmoid in profile view. This is flanked by two pairs of lateral cusplets also strongly lingually directed and well individualized. The main cusp and cusplets are united by fine but sharp and well-developed cutting edges running continuously. The outer pair of cusplets is about twice the size of the inner pair but all are equally slender. Crown ornament consists of rare vertical ridges on the labial face of the main cusp (two ridges) and outer cusplets (several ridges) that do not cover more than the lower third of the cusps. The lingual ornament consists of densely arranged and fine vertical ridges that are interrupted and slightly undulating. These are present on the main cusp and cusplets and do not reach the upper third of the cusps. The root is extremely thin and developed lingually (lingual torus). A medio-lingual bulge is present, devoid of foramina. Several foramina of variable sizes are present on both sides of the medio-lingual bulge, in the depressed marginal regions. The thin lingual root face is pierced by a wide median foramina and a pair of small foramina is present on the labial face below the contact between the inner and outer cusplet. The basal root face is fairly flat and pierced by various small foramina. Remarks The morphology presented by this tooth (sigmoid main cusp, two lateral cusplets with the outer pair being higher than the inner) is typical of cladodont sharks. Moreover, the small size of this tooth, slender main cusp, presence of a medio-lingual bulge and crown ornaments are combined characters that indicate affinities with Falcatidae (for example, Stethacanthulus , Denaea, Falcatus ). Although most representatives of this family possess teeth with a baso-labial projection (absent in the tooth described here), some derived forms such as Stethacanthulus meccaensis lack this character [4] . The family Falcatidae and order Symmoriiformes were thought to have gone extinct after the Cisuralian (Permian), some 130 myrs before the Valanginian. Resemblances with chlamydoselachid neoselachians are only superficial. In chlamydoselachids, the root is holaulacorhize, although the main axial groove is secondarily closed lingually. Chlamydoselachid teeth have diverging outer pair of cusplets projecting lingually and nearly as developed as the main cusp. They show a very different root morphology with two lingual projections separated by a marked V-shaped notch and corresponding axial groove on the lingual protuberance, no occlusal median convexity and a basal face showing a median labio-lingual crest with depressed marginal areas. Order Ctenacanthiformes Glikman, 1964 Ctenacanthiformes indet. ( Fig. 2f–j ) Material. One tooth (specimen VAL 54). Locality, horizon and age. Mas d’Antrigoule, (Gard County, Southern France); N. neocomiensis Zone, latest early Valanginian (Early Cretaceous). Description This tooth is of minute size and wider (less than 1 mm wide) than high. The main cusp is slightly inclined lingually and flanked by a pair of lateral cusplets (one is broken) in more labial position. Both the main cusp and cusplet show a convex lingual face and fairly flat labial face. The cutting edges are fine and interrupted between the main cusp and cusplet by a narrow notch. The lingual face of the main cusp and cusplet bear a pair of oblique marginal folds that follow the outline of the cutting edges. The labial crown face shows a strong basal depression at the base of the main cusp, semi-circular in labial view. The root is fairly high but with a reduced labial face, depressed and overhung by the crown in its centre. The lingual face is dominated by a pair of wide and high root protuberances situated on each side of the base of the main cusp. The developed medio-lingual region of the root is pierced by a wide foramen that is flanked by two pairs of smaller foramina. Other smaller foramina are present on the margino-lingual root faces. The basal root face appears fairly concave. Two slight baso-labial protuberances are present as well as a thin baso-lingual bulge that is developed along the lingual root edge. Remarks By the presence of a pair of margino-lingual and baso-labial protuberances, the root morphology of this tooth is similar to that of some Ctenacanthidae ( Glikmanius ) and to other ctenacanthiforms of unknown affinities ( Heslerodus, ‘Ctenacanthus’ costellatus ). Likewise, the crown morphology (flat labial crown face, medio-labial depression at the base of the crown) is identical to the above-mentioned ctenacanthiform genera, although the size of the tooth described here is closer to that of Heslerodus . The combined dental characters present in this specimen allow its attribution to the ctenacanthiform sharks. More material would be needed to identify this probably new taxon at lower taxonomic ranks. Teeth of last representatives of the order Ctenacanthiformes ( Heslerodus, Glikmanius ) were known from the Guadalupian (Permian). Cladodontomorphii indet. ( Fig. 2k–s ) Material. Four teeth (specimens VAL 55, 56, 57, 58). Locality, horizon and age. Mas d’Antrigoule, (Gard County, Southern France); N. neocomiensis Zone, latest early Valanginian (Early Cretaceous). Description Teeth of this taxon are wider than high and under 2 mm wide. The main cusp is smooth, biconvex and slightly inclined lingually. This bears well marked and sharp cutting edges strongly oblique near the base of the cusp in labial view. A pair of converging and triangular lateral cusplets is present, well individualized from the main cusp by notches separating the cutting edges. The lateral heels are high, sharp and oblique. The mesial heel is not or poorly separated from the cusplets by a slight notch. Distally, however, a notch more deeply separates the mesial cusplet from the heel, which thus resembles an additional cusplet. The heels are oriented lingually and taper before reaching the marginal root angles. The root is thin, mesio-distally elongate and fairly labio-lingually compressed. The basal root face is flat with the exception of the branch extremities that are bent basally. A pair of baso-labial root protuberances is present, situated below the base of the main cusp. The labial root face is very low and slightly flared. The lingual root face is well-developed and strongly projects lingually. A wide bulge occupies the majority of the lingual face except the lingual edge. The bulge is pierced by a wide median foramen with corresponding notch that opens lingually. Numerous additional foramina are also present on the lingual root face. Lateral teeth differ from anteriors by the distal inclination of the main cusp, whereas latero-posterior teeth are smaller, less mesio-distally developed with a more robust main cusp. Remarks Teeth of this taxon show combined features of various cladodontomorph shark groups. The lingual root face is more reminiscent of that of some Symmoriidae (for example, Stethacanthulus ), whereas the basal root face (pair of baso-labial protuberances) is more similar to that of some ctenacanthiform (for example, Glikmanius , Heslerodus ) or cladoselachiform taxa (for example, Cladoselache ). However, the peculiar crown morphology differs from that of representatives of cladodontomorphs and this taxon is thus left in open nomenclature within the Cladodontomorphii. Complementary enameloid analyses As a complement to the morphological identifications, we performed tooth enameloid microstructure analyses on two of the three Valanginian taxa described above as well as on a Permian cladodontomorph shark. Among the three enameloid layers (external shiny-layered enameloid (SLE); intermediate parallel-bundled enameloid (PBE); inner tangled-bundled enameloid), commonly present in teeth of neoselachian sharks (selachimorphs), only the PBE is considered the synapomorphy of this group [6] , [7] . This layer does not appear to be present in modern rays and skates (batoids) and in other stem chondrichthyan groups and hybodont sharks (which were claimed to have a single-layered enameloid in the vast majority of taxa studied, but see ref. 8 ). However, this assertion was based on extremely scarce data in comparison to the high stem chondrichthyan diversity and some of these rare analyses used section studies that do not allow clear identification of bundles [9] . We performed enameloid microstructure analyses on mid-Permian Ctenacanthiformes teeth of the species Neosaivodus flagstaffensis collected from the type locality in Arizona in order to test this hypothesis. Mid-Permian Ctenacanthiformes were chosen for this analysis because they are among the last representatives of the Palaeozoic Cladodontomorphii and their teeth did not suffer recrystallization as opposed to most Carboniferous stem Chondrichthyan fossil teeth. Surface etching performed on the single tooth of Ctenacanthiformes indet. ( Fig. 3a ) shows the presence of bundles of crystallites below a well-developed outer layer composed of individualized and randomly oriented crystallites. Parallel bundles (PBE) run apico-basally and change orientation near the cutting edge where they are perpendicular to its axis. It should be noted that the change in orientation occurs relatively far from the cutting edge’s axis. 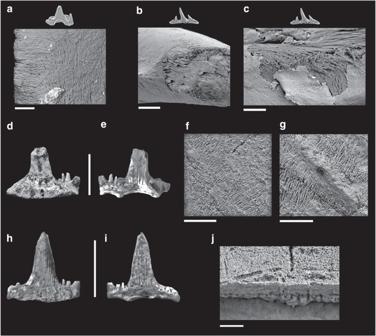Figure 3: Enameloid microstructure of Valanginian and Permian cladodontomorphs. (a) Surface etching of Ctenacanthiformes indet. VAL 54, showing parallel bundles of enameloid crystallites running apico-basally and changing orientation near the cutting edge (left). Scale bar, 30 μm. (b,c) Enameloid microstructure of Cladodontomorphii indet. (b) VAL 58, surface etching of the broken apex showing parallel bundles of enameloid crystallites (in ‘cross section’) running apico-basally and changing orientation near the cutting edge (left). Scale bar, 15 μm. (c) VAL 57, surface etching of the distal cutting edge near the apex showing bundles of crystallites running apico-basally and changing orientation near the cutting edge (oriented perpendicular to the latter). Scale bar, 5 μm. (d–j)Neosaivodus flagstaffensisfrom the mid-Permian of Arizona. (d–g) MHNG GEPI V5619, lateral tooth in (d) lingual and (e) labial views. Scale bar, 5 mm. (f) Surface etching of the distal area of the labial face showing parallel bundles of enameloid crystallites. Scale bar, 60 μm. (g) Surface etching of the distal area of the labial face showing parallel bundles of enameloid crystallites oriented perpendicular to the cutting edge (bottom left) below a labial fold. Scale bar, 60 μm. (h–j) MHNG GEPI V5648, anterior tooth in (h) lingual and (i) labial views. Scale bar, 5 mm. (j) Surface etching of the broken apex showing parallel bundles of enameloid crystallites (in ‘cross section’) below the shiny layered enameloid layer composed of individualized crystallites. Scale bar, 8 μm. Figure 3: Enameloid microstructure of Valanginian and Permian cladodontomorphs. ( a ) Surface etching of Ctenacanthiformes indet. VAL 54, showing parallel bundles of enameloid crystallites running apico-basally and changing orientation near the cutting edge (left). Scale bar, 30 μm. ( b , c ) Enameloid microstructure of Cladodontomorphii indet. ( b ) VAL 58, surface etching of the broken apex showing parallel bundles of enameloid crystallites (in ‘cross section’) running apico-basally and changing orientation near the cutting edge (left). Scale bar, 15 μm. ( c ) VAL 57, surface etching of the distal cutting edge near the apex showing bundles of crystallites running apico-basally and changing orientation near the cutting edge (oriented perpendicular to the latter). Scale bar, 5 μm. ( d – j ) Neosaivodus flagstaffensis from the mid-Permian of Arizona. ( d – g ) MHNG GEPI V5619, lateral tooth in ( d ) lingual and ( e ) labial views. Scale bar, 5 mm. ( f ) Surface etching of the distal area of the labial face showing parallel bundles of enameloid crystallites. Scale bar, 60 μm. ( g ) Surface etching of the distal area of the labial face showing parallel bundles of enameloid crystallites oriented perpendicular to the cutting edge (bottom left) below a labial fold. Scale bar, 60 μm. ( h – j ) MHNG GEPI V5648, anterior tooth in ( h ) lingual and ( i ) labial views. Scale bar, 5 mm. ( j ) Surface etching of the broken apex showing parallel bundles of enameloid crystallites (in ‘cross section’) below the shiny layered enameloid layer composed of individualized crystallites. Scale bar, 8 μm. Full size image Enameloid microstructure analyses made on two teeth of Cladodontomorphii indet. ( Fig. 3b,c ) show the presence of two distinct layers. The outer layer is composed of thin individualized crystallites randomly oriented. The inner layer is made of a typical PBE layer with apico-basally oriented bundles showing a low degree of compaction. Some superficial bundles of the PBE are oriented perpendicular to the cutting edge axis well away from the latter, and these superficial bundles make up the cutting edge’s thickness. No randomly oriented bundles were identified between the PBE and dentine. Study of the enameloid microstructure of two N. flagstaffensis teeth ( Fig. 3d–j ) revealed the presence of two distinct enameloid layers. The outer layer is reminiscent of the SLE with thin, randomly oriented and individualized crystallites. This layer is well-developed and also makes up the vertical labial folds ( Fig. 3g ). On the labial crown face, near the distal cutting edge and below the SLE are bundles of crystallites showing a low degree of compaction (similar to the PBE of the Valanginian taxa studied here) and an orientation perpendicular to the cutting edge. Further from the cutting edges, bundles are oriented apico-basally ( Fig. 3f ) and are in direct contact with the underling dentine ( Fig. 3j ). Exploration of the tooth enameloid microstructure of two taxa of the Valanginian cladodontomorph assemblage reported here (Ctenacanthiformes indet. and Cladodontomorphii indet.) shows the presence of crystallites associated into bundles (PBE). These are oriented apico-basally and parallel to the crown surface, a character considered restricted to modern shark tooth enameloid (Selachimorpha). However, enameloid study of mid-Permian unquestionable ctenacanthiform teeth ( N. flagstaffensis ) demonstrates that this feature is also present in stem chondrichthyans ( Fig. 3d–j ) and consequently not restricted to modern sharks. In addition, similarities in the enameloid microstructure of N. flagstaffensis and the two Valanginian taxa studied here (low compaction of the bundles of the PBE, absence of the underlying tangled-bundled enameloid layer) are noteworthy. The presence of a PBE in N. flagstaffensis also raises questions on the diagnostic feature of enameloid in elasmobranchs (the diversity in tooth morphologies and especially root features appear better surveyed) and on the settlement of the three-layered enameloid in selachimorphs, but this is beyond the scope of this research. Although the histological structure observed in teeth of N. flagstaffensis questions the monophyly of cladodontomorph sharks, it demonstrates that the histology of the Valanginian teeth is not incompatible with Palaeozoic sharks and thus reinforces the morphological-based identifications at taxonomic levels below Cladodontomorphii. Before this discovery, the last known unambiguous representatives of the superorder Cladodontomorphii (Symmoriiformes and Ctenacanthiformes, see refs 4 , 10 ) were Late Permian in age [4] , [11] , [12] , [13] . All allegedly Triassic cladodontomoph shark occurrences have been re-evaluated (for example, the Middle Triassic Acronemus tuberculatus [14] ) or have very dubious taxonomic values (Early Triassic fin spines [15] and denticles [16] ). It was thus considered that, with the exception of rare Early Triassic eugeneodontiforms [17] , no marine representatives of the stem chondrichthyans crossed the end-Permian mass extinction; the post-Permian chondrichthyans being euselachians (hybodont sharks and modern elasmobranchs), euchondrocephals (holocephals and relatives) and the freshwater xenacanthiform sharks. The Early Cretaceous occurrences reported here considerably extend the time range of Cladodontomorphii of circa 120 myrs, but also generate a gap in the fossil record of the group of equal duration ( Fig. 4 ). The recorded gap in the cladodontomorph lineage is almost 50% longer in duration than the gap observed in the coelacanth lineage, and represents the longest gap in the fossil record for an extinct marine vertebrate group. This gap took place after the largest mass extinction of the Phanerozoic [18] , [19] . Whereas Palaeozoic cladodontomorphs lived preferentially in neritic marine environments and, to a lesser extent, other shelf palaeohabitats [4] , [12] ( Table 1 ), the relatively diverse Early Cretaceous assemblage described here was found from outer platform deposits. This fossil record pattern, reminiscent of that observed in the coelacanth lineage from the Late Cretaceous onwards ( Table 1 ), indicates that some cladodontomorph groups may have survived the end-Permian and the subsequent Triassic-Jurassic mass extinction events by occupying refuge environments. As for Cainozoic coelacanths, the absence of Triassic and Jurassic cladodontomorphs is due to the scarcity of known deep-sea vertebrate assemblages from this time interval. Whereas the Triassic-Jurassic event had a visible impact on fish diversity [20] , [21] , [22] , [23] , the dramatic aftermaths of the Permo-Triassic event on fish groups remain poorly understood [2] . Regardless of the nature of the events that affected the Earth system at the Permo-Triassic boundary (widespread anoxia in shallow marine settings [24] , [25] , [26] , [27] , ocean acidification [28] , [29] , perturbations of the global carbon cycle [30] and global warming [31] ), the stable outer shelf and deep-sea environments may have represented refuge zones in contrast to more exposed neritic habitats. 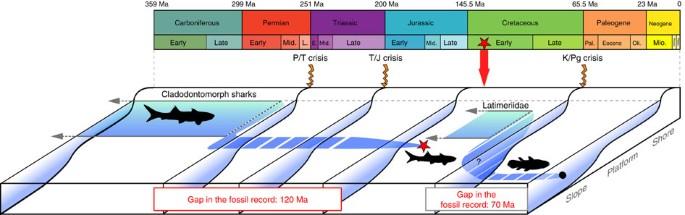Figure 4: Stratigraphic comparison of the cladodontomorph and latimeriid fossil record and palaeohabitat distribution. Previous (Palaeozoic) occurrences of cladodontomorphs were from all shelf habitats albeit mainly near-shore, whereas the occurrence reported here is from outer platform environment and expands this group’s stratigraphic range to circa 120 million years. Red star refers to the finding reported in this paper. P/T crisis, Permo/Triassic crisis; T/J crisis, Triassic/Jurassic crisis; K/Pg crisis, Cretaceous/Palaeogene crisis; Ma, mega-annum. Figure 4: Stratigraphic comparison of the cladodontomorph and latimeriid fossil record and palaeohabitat distribution. Previous (Palaeozoic) occurrences of cladodontomorphs were from all shelf habitats albeit mainly near-shore, whereas the occurrence reported here is from outer platform environment and expands this group’s stratigraphic range to circa 120 million years. Red star refers to the finding reported in this paper. P/T crisis, Permo/Triassic crisis; T/J crisis, Triassic/Jurassic crisis; K/Pg crisis, Cretaceous/Palaeogene crisis; Ma, mega-annum. Full size image Table 1 Stratigraphic and paleoenvironmental ranges of the taxa considered. Full size table Habitat shifts have been observed for fish clades surviving the Hangenberg event at the Devonian/Carboniferous boundary (for example, gyrancanthid acanthodians, rhizodonts [2] ). Other examples of deep-sea environments identified as momentary refuges are known for invertebrates [32] , [33] and conodonts [34] . In most of these cases, however, the retreat is followed by repopulation of shallower environments during a recovery phase, which induces, if any, short gaps in the fossil records. The long-lasting hostile environmental conditions in the post-Permian neritic habitats may have precluded repopulation [35] and probably led to the permanent settlement of some cladodontomorph sharks in deeper waters during the early Mesozoic. The gap in the cladodontomorph fossil record reported here is the longest ever recorded for a marine vertebrate lineage and is caused by the poor representation of deep marine environments in the sedimentary record. A comparable instance, although of shorter gap duration ( Table 1 ), is the carpertshark Orectoloboides (‘mid’-Cretaceous to Eocene, ca 60 myrs). This genus crossed the Cretaceous/Paleogene boundary and shifted from neritic to deep-sea habitats [36] , thus indicating that the fossil record patterns reported here are more common among marine fishes than previously expected. The discovery of both living Latimeria species in 1938 and 1998 revealed that relatively deep-sea habitats may serve as refuge for representatives of ancient fish lineages. This emphasises the refugial role deep-sea environments may have played during most of the evolutionary history of marine vertebrates. The scarcity of deep-sea deposits yielding vertebrate remains, however, obscures large parts of the evolution of palaeobiodiversity of which a new piece is unveiled here. Sediment processing About 500 kg of sediment were sampled, processed and sorted. Bulk-sampled rocks were then acid processed using diluted 10% acetic acid and fossil remains were picked from residues that were formerly sieved down to a fine mesh size (350 μm). About 10,000 identifiable teeth were recovered and among them, only those belonging to the species Welcommia bodeuri have been studied and described in details so far [37] . The remaining fauna is dominated in both taxonomic richness and number of specimens by hexanchiforms (cow sharks), thus confirming the fairly deep paleoenvironmental settings. Elasmobranch remains (teeth, scales and vertebrae) represent the largest part of the fossil material recovered. Enameloid microstructure analyses Exploration of tooth enameloid microstructure was carried out using acid etching of tooth surfaces. This method was chosen because the enameloid layer considered as one of the synapomorphies of neoselachian sharks (PBE) is more clearly observable using surface etching and because Valanginian specimens are scarce and delicate preventing the use of destructive section studies. Surface etchings using 10% HCl (during 10 s.) were made on enameloid breaks over tooth surfaces and broken crown apices so that ‘section’ views were possible. Surface studies were made on the following Valanginian taxa: Ctenacanthiformes indet. (on the single tooth, VAL 54) and Cladodontomorphii indet. (VAL 57 and VAL 58). The single tooth corresponding to Falcatidae indet. could not be etched because of the minute size, preservation and absence of breaks on this specimen. In order to test the validity of the PBE as a synapomorphy of neoselachian sharks (Selachimorpha), the enameloid microstructure of unquestionable ctenacanthiform teeth was explored. Surface etching was carried out on teeth of Neosaivodus flagstaffensis . This material comes from the type locality (Kachina Microsite, lower Fossil Montain Member, Kaibab Formation) latest Cisuralian/early Guadalupian in age (see ref. 38 ). Specimen repository Figured Valanginian specimens (VAL 36, 54–58) are housed in the collections of the Paleontology Department, University of Montpellier 2 (Institut des Sciences de l’Evolution de Montpellier) and Permian specimens from Arizona (MHNG GEPI V5619 and MHNG GEPI V5648) are housed in the collections of the Natural History Museum of Geneva. How to cite this article: Guinot, G. et al. Cretaceous stem chondrichthyans survived the end-Permian mass extinction. Nat. Commun. 4:2669 doi: 10.1038/ncomms3669 (2013).